Evidence of superdense aluminium synthesized by ultrafast microexplosion At extreme pressures and temperatures, such as those inside planets and stars, common materials form new dense phases with compacted atomic arrangements and unusual physical properties. The synthesis and study of new phases of matter at pressures above 100 GPa and temperatures above 10 4 K—warm dense matter—may reveal the functional details of planet and star interiors, and may lead to materials with extraordinary properties. Many phases have been predicted theoretically that may be realized once appropriate formation conditions are found. Here we report the synthesis of a superdense stable phase of body-centred-cubic aluminium, predicted by first-principles theories to exist at pressures above 380 GPa. The superdense Al phase was synthesized in the non-equilibrium conditions of an ultrafast laser-induced microexplosion confined inside sapphire ( α -Al 2 O 3 ). Confined microexplosions offer a strategy to create and recover high-density polymorphs, and a simple method for tabletop study of warm dense matter. Ordinary substances behave in extraordinary ways at high temperature and pressure, resulting in completely new phases of matter [1] , [2] , [3] , [4] , [5] , [6] . This type of matter regulates processes deep in the Earth as well as in the cores of other planets [1] , [7] , [8] . The quest to simulate these conditions, and study the behaviour of materials under extreme pressure and temperature has a long history [9] , with a dramatic advance in this direction being made by the invention of diamond anvil cell [10] . During the last century, pressure and temperature records have increased continuously, and it is now possible to obtain multimegabar static pressures, with simultaneous heating by laser up to 3,000 K (refs 1 , 5 , 11 , 12 ). In fact, recently, conditions at the Earth's core of 364 GPa and 5,500 °C were recreated in the lab [13] . Even more extreme but transient high-pressure/-temperature conditions have been created by dynamic methods using explosives and megajoule-class lasers [14] , [15] , [16] , [17] , [18] , [19] . It has been predicted that new classes of materials with unusual combinations of physical properties should exist under conditions of extreme pressure and temperature [4] , [20] , [21] , [22] . For instance, high-pressure structural behaviour of crystalline metallic Al phases has been the subject of first-principles theoretical studies [20] , [23] , [24] , which predict a sequence of phase transitions with estimated static transition pressures within the 120–360 GPa and 200–560 GPa ranges for fcc hcp (face-centred-cubic to hexagonal-close-packed) and hcp bcc transitions, respectively. However, only the existence of hcp-Al phase has been confirmed experimentally so far [22] , [25] . Prediction of aluminium phases at terapascal pressures has been reported [26] but could not be validated by state-of-the-art high-pressure synthesis methods. Recently, it was demonstrated that it is possible to create extreme pressure and temperature conditions in table-top laboratory experiments with ultrashort laser pulses focussed inside a transparent material, with intensity in the focal spot significantly above the threshold for optical breakdown [27] , [28] , [29] . Tight focusing of a ~100-fs laser pulse with 100 nJ energy deep inside a crystal, deposits an energy density of several MJ cm −3 into a submicron volume, several times higher than the strength of any material. This causes the solid to superheat and form a plasma. The confined plasma explodes and generates a powerful shock wave that expands out of the focal volume and compresses the surrounding pristine material [27] , [28] , [29] . The shock wave of the expanding plasma can reach pressures of over 10 megabar (1 TPa), triggering dramatic changes in the material properties. One of the essential novelties of the new method is that the modified material remains confined in a strongly localized region inside a bulk of pristine crystal, and can be investigated later. Here we report on the synthesis of a new stable high-pressure phase, bcc-Al, formed by ultrafast laser-induced microexplosion confined inside sapphire α -Al 2 O 3 (refs 28 , 29 ). The phase is preserved inside the amorphous compressed sapphire produced from a hot, dense, non-equilibrium and short-lived plasma. We suggest that the sapphire constituents, aluminium and oxygen, become spatially separated in the hot expanding plasma because of the differences in the ion diffusion velocity, and a new bcc-Al phase is 'frozen' within the compressed sapphire. Synchrotron X-ray diffraction microanalysis ( μ XRD) shows that the diffraction peaks observed in our sample perfectly match the bcc-Al structures predicted to exist at high pressures [20] , [23] , [24] . Formation of voids In our experiments, we irradiated α -Al 2 O 3 (corundum, a variety of sapphire) crystals with 150-fs laser pulses focused at depths of several micrometers, using a high numerical aperture microscope lens (Methods). Sapphire has a very large bandgap of 9.8 eV, and is of technological importance, given that it is a high-hardness ceramic material with a high bulk modulus of B =239–257 GPa (ref. 30 ), and because the void inside sapphire is well distinguishable by an optical contrast and well defined when compared with softer materials such as silica or polystyrene. Laser radiation caused the formation of voids with compressed shells within the sapphire crystal ( Fig. 1 ). The size of the voids and the compressed-shell thickness were measured using transmission and scanning electron microscopes (TEM & SEM) after opening the enclosed laser-affected zone by Focused Ion-beam milling. The average radius of the combined void and shell structures was ~360 nm, twice as large as the shell thickness of ~180 nm. Assuming conservation of mass, the average shell density was δ =1.14 ρ s =4.54 g cm −3 , where ρ s =3.98 g cm −3 is the initial density of sapphire. This shell was identified as amorphous material by TEM and chemical etching because amorphous sapphire has a much higher solubility in hydrofluoric acid than crystalline sapphire [28] . 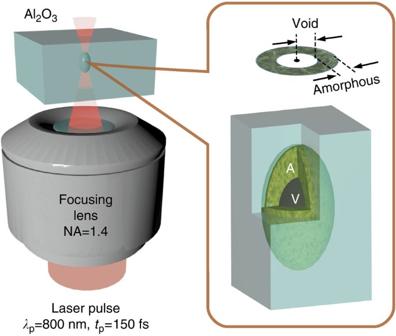Figure 1: The method to create high-density phase by the ultrashort laser pulse triggered and spatially confined microexplosion. A tightly focused femtosecond pulse generates hot plasma in sapphire, which in turn produces a strong shock wave, which compresses the material against the surrounding pristine Al2O3crystal into a densified amorphous phase A and forms a void V in the centre of a laser-induced microexplosion. The superdense bcc-Al phase was found within this compressed material. Figure 1: The method to create high-density phase by the ultrashort laser pulse triggered and spatially confined microexplosion. A tightly focused femtosecond pulse generates hot plasma in sapphire, which in turn produces a strong shock wave, which compresses the material against the surrounding pristine Al 2 O 3 crystal into a densified amorphous phase A and forms a void V in the centre of a laser-induced microexplosion. The superdense bcc-Al phase was found within this compressed material. Full size image Samples for μ XRD analysis were prepared by making regular 3D arrays of laser-modified areas with a period of 2 μm within a region of (50×50×70) μm 3 in polished slabs of α -Al 2 O 3 . μ XRD characterization of the laser-processed region was carried out using a monochromatic 33 keV ( λ =0.3757 Å) X-ray beam with a cross-section of 5×10 μm at full width half maximum (FWHM). The microfocused X-ray beam was oriented axially, approximately parallel to both the original laser beam and to the crystallographic z-axis of the sapphire, and was scanned in 10 μm steps over both patterned and non-patterned regions. 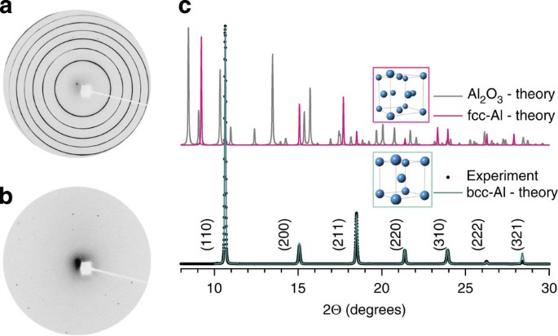Figure 2: Evidence of bcc-Al formation within the laser structured regions. Micro-X-ray diffraction (μXRD) image acquired (a) in the centre of the shockwave compressed area, and (b) outside the shockwave compressed area. (c) Comparison between a radially integrated experimentalμXRD profile obtained from the experimental data shown in (a), and theoreticalμXRD profile expected for bcc-Al refined using Materials Studio package, assuming 18 nm crystalline size. The crystalline (hkl) plane indices are shown next to the peaks. For comparison, simulated profiles of host sapphire (vertically offseted grey) and native fcc-Al (purple) are also shown. Evidence of a superdense phase of Al Figure 2a,b show 2D μ XRD images collected at laser-modified and intact areas in the sample. There are pronounced diffraction rings in the modified regions, whereas pristine regions show only a background of single-crystal-like sharp spots. An azimuthally-integrated μ XRD pattern of Figure 2a was thoroughly compared with the X-ray Bragg peak positions of known and theoretically predicted high-pressure Al 2 O 3 phases [31] , and for all possible Al-O compounds at various combinations of density and temperature, but no satisfactory match was obtained. Also, given the large difference in electronegativity at high pressure [32] and in the atomic radii [33] of Al and O, a solid solution of Al and O cannot explain the observed μ XRD spectra, as may be seen from the empirical Hume–Rothery analysis [34] outlined in the Methods. Further examination revealed that the measured peak positions could be perfectly indexed as a bcc-Al structure (space group Im-3m) with a lattice constant a =2.866 Å (11.77 Å 3 per atom), which matches a predicted [20] , [23] , [24] , but not yet experimentally observed, high-pressure Al phase; this bcc-phase is 41% more dense than the native fcc-phase of Al; the density of bcc-Al ρ bcc =1.41× ρ fcc =3.81 g cm −3 . Figure 2c shows a comparison between the experimental μ XRD pattern and Rietveld-refined profile of bcc-Al. 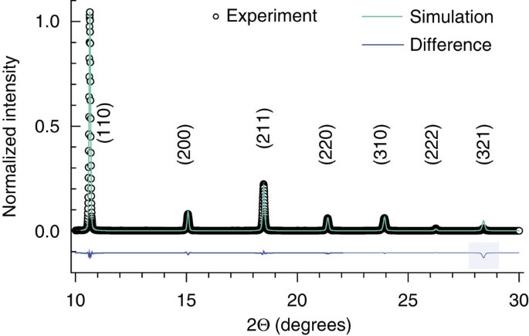Figure 3: Rietveld refinement profile of the bcc-Al structure. A difference curve is plotted for comparison with offset. The last Bragg peak intensity was not included in the fit, because only a fraction of the diffraction ring was acquired in the XRD image (enclosed in a shaded-box). The refinement fit is shown together with experimental in Figure 3 . Shapes of the Bragg peaks were fitted using Rietveld refinement with crystallite size and microstrain as fitting parameters, yielding a crystallite size of 17.9 nm and strain of 0.26%, closely matching the values calculated using Scherrer's algorithm [35] : L = Kλ /( β cos θ ), where L =18±2 nm is the size of the nanocrystallite, K =0.891 is a constant, β is the FWHM of the diffraction peak, and θ is the diffraction angle. Figure 2: Evidence of bcc-Al formation within the laser structured regions. Micro-X-ray diffraction ( μ XRD) image acquired ( a ) in the centre of the shockwave compressed area, and ( b ) outside the shockwave compressed area. ( c ) Comparison between a radially integrated experimental μ XRD profile obtained from the experimental data shown in ( a ), and theoretical μ XRD profile expected for bcc-Al refined using Materials Studio package, assuming 18 nm crystalline size. The crystalline (hkl) plane indices are shown next to the peaks. For comparison, simulated profiles of host sapphire (vertically offseted grey) and native fcc-Al (purple) are also shown. Full size image Figure 3: Rietveld refinement profile of the bcc-Al structure. A difference curve is plotted for comparison with offset. The last Bragg peak intensity was not included in the fit, because only a fraction of the diffraction ring was acquired in the XRD image (enclosed in a shaded-box). Full size image Indexing of the μ XRD pattern revealed that the observed Bragg peaks originate from a material having bcc unit cells with a lattice constant a =2.866 Å and space group Im-3m (229). Such unit cells have only two unique atoms at atomic coordinates of (0, 0, 0) and (1/2, 1/2, 1/2). Hence, the two shortest interatomic distances are 2.482 Å (between the corner and centre atoms) and 2.866 Å (between the corner atoms). As microexplosions were confined in the bulk of crystalline Al 2 O 3 , the only constituents that can contribute to the observed Bragg peaks are Al and O. The shorter interatomic distance agrees well with a double atomic radius of Al of 1.25 Å (ref. 36 ), thus suggesting Al–Al bond. Because the atomic radius of oxygen is much smaller, 0.6 Å, the length of Al–O bond would be about 1.85 Å. For instance, bonds of similar length can be found in a crystalline Al 2 O 3 lattice, where the two shortest interatomic distances are 1.852 Å and 1.975 Å (˚ http://www.icdd.com/ ). In our bcc lattice, the presence of Al–O bond would result in a μ XRD pattern drastically different from the one observed. Hence, oxygen cannot form bonds with aluminium in the identified bcc structure with a =2.866 Å, and does not contribute to the experimental μ XRD pattern shown in Figure 2c . Consequently, both atoms in the bcc unit cell are Al, and the observed μ XRD pattern is due to nanocrystallites of pure aluminium. 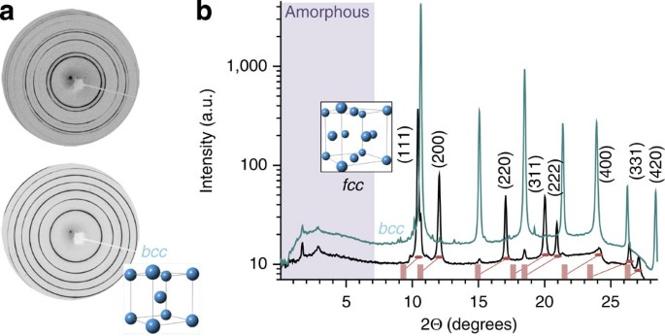Figure 4: Determination of the residual pressure in the vicinity of the retrieved bcc- and fcc-Al nanocrystallites. (a) Micro-X-ray diffraction (μXRD) patterns from the laser-structured region (the pattern ofFigure 2) where bcc-Al signatures or fcc-Al are dominant. (b) Comparison of the two integratedμXRD patterns shown in (a). Numerical fit of the experimentally observed peaks by the fcc-Al structure with a cell size ofa=3.584 Å is achieved; bottom purple marks show the expected position of the fcc-Al peaks at room conditions witha=4.049 Å. The retrieved fcc-Al is subjected to pressures ~60–100 GPa (seeMethodsfor details). The μ XRD provides a non-destructive verification of the new bcc-Al phase which is stabilized in a compressed enclosure, as estimated by an observed co-existence of bcc- as well as a ~60 GPa-compressed fcc-Al phase as deduced from a shift of μ XRD peaks shown in Figure 4 (Methods). Figure 4: Determination of the residual pressure in the vicinity of the retrieved bcc- and fcc-Al nanocrystallites. ( a ) Micro-X-ray diffraction ( μ XRD) patterns from the laser-structured region (the pattern of Figure 2 ) where bcc-Al signatures or fcc-Al are dominant. ( b ) Comparison of the two integrated μ XRD patterns shown in ( a ). Numerical fit of the experimentally observed peaks by the fcc-Al structure with a cell size of a =3.584 Å is achieved; bottom purple marks show the expected position of the fcc-Al peaks at room conditions with a =4.049 Å. The retrieved fcc-Al is subjected to pressures ~60–100 GPa (see Methods for details). Full size image Spatial separation of ions The observed formation of crystalline aluminium out of aluminium oxide is experimental evidence of a quite unusual and unexpected phenomenon, namely spatial separation of oxygen and aluminium ions in conditions of complete confinement and preserved stoichiometry. We propose the following explanation for this effect. Ultrashort laser pulses with intensity above the optical breakdown threshold break bonds of Al 2 O 3 and ionize the constituent atoms into plasma, which exists until the material cools down below the thermal ionization threshold. While this plasma exists, the Al and O ions diffuse and scatter at different rates, allowing spatial separation of the sapphire constituents ( Fig. 5 ). 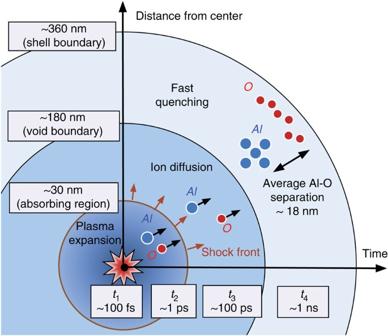Figure 5: Synthesis of materials via spatial separation of elements in the plasma state. Schematic explanation of spatial and temporal transformations in the volume of ionized sapphire affected by a microexplosion, leading to spatial separation of Al and O ions and quenching of the bcc-Al. Horizontal and vertical axes represent time and distance from the centre of microexplosion, respectively. Figure 5: Synthesis of materials via spatial separation of elements in the plasma state. Schematic explanation of spatial and temporal transformations in the volume of ionized sapphire affected by a microexplosion, leading to spatial separation of Al and O ions and quenching of the bcc-Al. Horizontal and vertical axes represent time and distance from the centre of microexplosion, respectively. Full size image The Rutherford cross-section, governs the Coulomb scattering of ions in plasma; here Z 1 and Z 2 are ion charges, is the reduced mass of the interacting particles, and ( v 1 − v 2 ) is their relative velocity [37] . The mean free path of the ions increases with the interaction energy. Hence, the mean free path becomes larger than the inter-atomic distance at a certain threshold energy level, around 10 eV in our experiments. The difference between the scattering and the diffusion length of ions with different masses becomes apparent above the threshold. This effect is especially pronounced in collisions of particles with significantly different masses. The maximum difference occurs in the case of electron–ion collisions, where the smallest mass is equal to the mass of a single electron [37] . The difference in the diffusion length between oxygen and aluminium ions leads to spatial separation that depends on the ion charge, mass and the rate of electron-to-ion energy transfer as estimated below. In a neutral solid, spatial separation of O and Al is physically impossible even when the molecular bonds are broken at elevated temperature, because the diffusion is insufficient to move atoms for a distance larger than the inter-atomic spacing. The major reason is that the cross-section for atomic collisions of neutral atoms is temperature independent. By contrast, collisions of ions in hot plasma are governed by the Rutherford cross-section, which is inversely proportional to the squared relative energy and reduced mass of the interacting particles [37] . The electron-to-ion energy transfer time in plasma is directly proportional to the ion's mass: ; here is the electron-phonon momentum exchange rate. Thus, the difference in mass becomes important at the early stage of plasma formation: the lighter O ions are heated more, gain more energy, and diffuse faster than the heavier Al ions. As a result, a unique non-equilibrium three-temperature state is established. The difference between the diffusion lengths leads to spatial separation of Al- and O-ions. The diffusion length and diffusion velocity D d = l mpf v ion /3 is expressed through the mean free path l mfp and velocity v i on of the ion. Diffusion continues during the time t d until the plasma temperature drops below a certain level. Thus, the separation distance between Al- and O-ions can be expressed in the following form: At a fixed temperature, the differences in the ions' velocity, mean free path, and diffusion length are related to the difference in their mass. The ratio of oxygen to aluminium ion velocity is expressed through the difference in mass as: ν O / ν Al =( M Al / M O ) 1/2 =1.3, consequently, the spatial separation can be expressed as follows: we assume here that each ion diffuses in plasma with the average ion mass M av =20 a.u. and μ Al, O = M Al, O M av /( M Al, O + M av ). One can see that the diffusion length of oxygen should exceed 100 nm to form the tens-of-nm sized crystallites observed in the experiments. Let us now estimate the diffusion coefficient of oxygen and the diffusion time t d , which define the diffusion length. The Coulomb collision cross-section for the temperature range of 10–50 eV only slightly exceeds the atomic cross-section. It is around σ R ≈10 −15 cm 2 . Therefore, the mean free path in solid density plasma is comparable to the interatomic distance. The lifetime of the plasma limits the ion separation period. Thermal ionization by electron impact continues the ionization process after the pulse almost at the same level as during the pulse, because the plasma temperature is much higher than the ionisation potential [29] . Therefore, plasma exists until cooling processes due to energy dissipation in the expanding shock wave and heat conduction reduce the temperature below the threshold of ≈10 eV. The process of void formation by rarefaction wave maintains the high temperature of ions in the central parts of the laser-affected volume. The density decrease in the central part of a spherical explosion is accompanied by an increase in temperature, keeping the pressure almost evenly distributed over the space of the central region [37] . The ion's mean free path is inversely proportional to the plasma density. According to hydrodynamic simulations of microexplosions [29] , mass density at the centre is around 0.1 g cm −3 at 0.9 ns after the microexplosion. Hence, the mean free path of oxygen ions moving away from the rarefied central area is within several nanometers, and their diffusion rate is around D d O ≈0.1 cm 2 s −1 . Taking the cooling time t d ≈1 ns in accordance with computer simulations [29] , the oxygen diffusion length is L d O ≈100 nm. Thus, separation of oxygen and aluminum ions in hot and dense plasma due to the difference in the diffusion rates appears to be a viable process (see equation (1)) responsible for the formation of superdense bcc-Al crystals. To conclude, this study shows that a femtosecond laser-induced microexplosion confined inside sapphire leads towards synthesis of a new and previously unobserved dense bcc-Al phase, which survives in a compressed state after fast quenching. The route of synthesis is via spatial separation of Al and O ions in short-lived hot non-equilibrium plasma of solid state density. We have demonstrated that high energy density produced in a simple tabletop experiment makes it possible to form an exotic high-density material phase, which could not be produced by other means. The mechanism responsible for the formation of the new phase of material can occur in a wide range of other materials that could be similarly subjected to extreme pressure and temperature conditions and converted into spatially confined plasma. As ultrafast lasers can operate at very high repetition rates within the MHz-range and deliver a high pulse energy [38] , laser-induced microexplosions offer a new strategy for the synthesis of high-pressure phases of materials in useful amounts in table-top laboratory conditions. Laser modification of sapphire The laser source was a Hurricane X (Spectra Physics) regeneratively amplified Ti:Sapphire femtosecond laser system, operating at a wavelength of 800 nm and producing pulses with a temporal length of about 150 fs. The pulses were focused in the sample using an oil-immersion objective (Olympus) with numerical aperture NA=1.4. The pulse energy in the focal spot was 135±6 nJ, corresponding to a peak intensity of I 0 =487 TW cm −2 . The sample, an 80 μm-thick sapphire slab (Shinkosha), was mounted on a high-precision three-dimensional translation stage controlled by piezoelectric transducers (Physik Instrumente). The stage was translated between consecutive laser shots along a predefined trajectory, such that an ordered pattern of void-structures was produced in the slab. The focusing depth below the surface of the sapphire sample was within the range 20–60 μm. Precompensation of the pulse group-velocity dispersion in the microscope lens and other optical elements along the optical path was done to ensure the shortest pulse duration at the focus. X-ray diffraction experiments and data processing μ XRD characterization of the laser-processed region was carried out by angle-dispersive X-ray microdiffraction at HPCAT beamline 16-BM-D of the Advanced Photon Source, Argonne National Laboratory. The monochromatic X-ray beam with energy of 33 keV ( λ =0.37571 Å) delivered by a Si (111) monochromator was focused by a pair of Kirkpatrick-Baez mirrors down to an area of (5.0×10.0) μm 2 (width×height), estimated at FWHM. X-ray diffraction patterns were collected in the transmission mode using a Mar345 Image Plate with typical exposure time per image of 50–100 s. The sample-to-detector distance and detector tilts were calibrated with a CeO 2 (NIST) standard. All two-dimensional μ XRD images were integrated to one-dimensional diffraction patterns using FIT2D software. Theoretical powder X-ray diffraction patterns expected for fcc-Al, bcc-Al, sapphire and high-pressure AlO x phases were calculated using the Materials Studio package (Accelrys). XRD pattern analysis, structure determination and Rietveld refinement was performed using X'Pert HighScore Plus (PANalytical) and Materials Studio (Accelrys) software. By indexing the X-ray diffraction pattern, we unconditionally identified the size and symmetry of the unit cell. The ability to observe seventh peak in the μ XRD pattern enabled us to avoid ambiguity and distinguish simple cubic and bcc structures. The unit cell obtained is body-centred-cubic with the unit cell parameter a =2.866 Å and space group Im-3m(229). The peak widths and intensities were fitted using Rietveld refinement. Peak shapes were fitted using crystallite size and strain as fitting parameters. This resulted in a crystallite size of 17.9 nm and strain of 0.26%. The resulting Rietveld refinement profile of the bcc-Al phase is shown in Figure 3 . The last Bragg peak intensity was not included in the fit, because only a fraction of the diffraction ring was acquired in the μ XRD image. The R-indices of the criteria of fit are R wp =0.08 and R p =0.05, which represent a high-quality fit for compounds with high symmetry. The major μ XRD peaks ride on a weak broad background, which also features many small peaks. This background is emphasized in the plot in Figure 4 . The broad background feature at small diffraction angles ( Fig. 4 ) originates from amorphous sapphire created by microexplosions, whereas the sharp not-Al-related peaks most likely originate from oxygen-rich AlO x phases as well as damaged and misoriented Al 2 O 3 regions. The fcc-Al phase was also present in the laser-affected region. μ XRD spectra revealed the presence of compressed fcc-Al diffraction peaks in several void-and-shell structures (see Fig. 3 ). The set of the diffraction peaks corresponding to fcc-Al and bcc-Al are compared in Figure 3b . As it can be seen, the fcc-Al pattern belongs to the space group Fm-3m (225) ( http://www.icdd.com/ ), the same as that for fcc-Al at the ambient conditions. However, the atomic volume of observed fcc-Al, V =11.51 Å 3 , is 1.44 times smaller than the volume of fcc-Al in the ambient conditions, V 0 =16.62 Å 3 . Thus, in our experiments fcc-Al is compressed practically to the same density as the newly born bcc-Al. The Young modulus of aluminium at room temperature comprises 70 GPa. An increase in density would result in a rise of the Young modulus up to 100 GPa. We estimate cautiously that residual pressure that will keep compressed fcc-Al inside a sapphire matrix is in the range 60–100 GPa (ref. 22 ). Therefore, one may expect residual strain to exist in the laser-compressed shell where fcc-Al and high-density bcc-Al were observed. Hume-Rothery analysis of Al and O solid solution The XRD profile comparable to that of bcc-Al can also be generated by a bcc unit cell of a substitutional alloy of Al and O with the same lattice constant a =2.866 Å. In the case of Al and O occupying distinct bcc lattice sites, owing to dissimilar scattering factors of Al and O, XRD pattern will exhibit Bragg peaks such as (111), (201), (122), (003), (113) and (203) within 2 θ =10–30° that are otherwise forbidden in bcc crystal structure. As these peaks are not present in the experimental XRD pattern shown in Figure 2 , we therefore exclude the existence of ordered Al-O alloy phase in our sample. The Bragg peak positions and relative intensities will match those of pure bcc-Al only, if both atomic sites of the bcc unit cell are randomly occupied by Al and O and with the same Al/O ratio, similarly to the case of Ce and Al [39] . The formation of such solid solution, however, has to satisfy empirical Hume–Rothery rules, which state that the atomic radii of the solute and the solvent must not differ by more than 15% and that their electronegativity should be within 0.4 of each other [34] . To calculate atomic radii of Al and O we use the phenomenological equation of state (EoS) by Vinet et al . [40] : where B 0 is the bulk modulus, B ′ 0 is pressure derivative of the bulk modulus, V 0 is the initial and V is the high-pressure phase volumes, respectively. We calculate atomic radii of Al and O at two pressures: 100 GPa—the estimated maximum remnant pressure of bcc-Al in Al 2 O 3 matrix after the laser pulse and 275 GPa—the theoretically predicted pressure for bcc-Al formation [41] . Following the EoS obtained by Akahama et al . [22] , we estimate atomic radii of bcc-Al as 1.189 and 1.087 Å, at pressures 100 and 275 GPa, respectively. To form solid solution with Al, oxygen has to be in a monatomic phase with atomic radii within 15% of that of Al. However, up to this date, no monatomic phase of solid oxygen has been experimentally observed up to pressures of 116 GPa (refs 42 , 43 ) and therefore experimental EoS for monatomic oxygen does not exist. Moreover, it has been predicted by Oda et al . [44] that molecular (diatomic) oxygen phase is stable over a wide range of pressures 100–2,000 GPa. The high stability of diatomic oxygen up to very high pressures makes it very unlikely that substitutional Al-O alloy can be formed. Nevertheless, some theoretical work has been done to predict monatomic solid oxygen phase and estimate its atomic radius at high pressures [44] , [45] , [46] . In the work by Anderson et al . [45] EoS of Fe oxides, corrected to remove the effects of Fe, was used. They estimated an atomic radii of monatomic oxygen at pressures 136, 330 and 360 GPa to be 0.94, 0.89 and 0.88 Å, respectively [45] . Because elements in many groups of the periodic table under high pressure exhibit similar sequence of structural phase transitions, further theoretical predictions utilized the fact that other group VIa elements, S, Se and Te, do form monatomic phases at high pressures [46] , [47] , [48] , [49] , [50] , [51] such as β -Po rhombohedral phase, which can be considered as simple cubic (sc) phase that is deformed along [111] direction. According to the band structure calculations performed by Suzuki et al . [46] , the most stable β -Po unit cell shape of monatomic solid oxygen is when c / a =1.04, where c and a lattice constants refer to the hexagonal setting [46] . Using this result and applying EoS obtained for molecular oxygen [42] , we estimate radius of monatomic solid oxygen in β -Po crystal structure as 0.906 and 0.827 Å for pressures 100 and 275 GPa, respectively. These values are in good agreement with the atomic radii reported by Anderson et al . [45] The atomic radii difference between Al (solvent) and O (solute) at pressures 100 and 275 GPa are 24% and do not satisfy HR rules for solid solution formation. Following the trend of group VIa elements, one can predict a formation of bcc-O crystal structure at even higher pressures [22] , [50] . Monatomic oxygen in such structure will display atomic radii of 0.986 and 0.902 Å at pressures 100 and 275 GPa, respectively. For the bcc-Al and bcc-O structures, the difference in atomic radii is 17%, too great to satisfy HR rules. The electronegativity can be calculated as EN =0.31×( Z +1)/ r c +0.5 (ref. 52 ), where Z is the valence electron numbers (3 and 6 for Al and O, respectively) and r c [Å] is the covalent radius. Assuming bcc-Al as a covalently bonded material, the estimated electronegativities for Al are 1.543 and 1.641 at pressures 100 and 275 GPa, respectively. Considering that monatomic oxygen in β -Po and bcc crystal structures is also covalently bonded, we can get the following electronegativites for O: β -Po structure—2.896 and 3.125, bcc structure—2.700 and 2.906 at 100 and 275 GPa pressures, respectively. The differences in electronegativities between Al and O are much larger than 0.4 for all estimated structures and therefore do not satisfy HR rules for solid solution formation either. On the basis of XRD data analysis and estimates of atomic radii and electronegativities, we conclude that solid solution of Al and O cannot be formed. How to cite this article: Vailionis, A. et al . Evidence of superdense aluminium synthesized by ultrafast microexplosion. Nat. Commun. 2:445 doi: 10.1038/ncomms1449 (2011).